Serotonergic neuronal death and concomitant serotonin deficiency curb copulation ability ofDrosophila platonicmutants Drosophila platonic ( plt ) males court females, but fail to copulate. Here we show that plt is an allele of scribbler ( sbb ), a BMP signalling component. sbb knockdown in larvae leads to the loss of approximately eight serotonergic neurons, which express the sex-determinant protein Doublesex (Dsx). Genetic deprivation of serotonin (5-HT) from dsx -expressing neurons results in copulation defects. Thus, sbb + is developmentally required for the survival of a specific subset of dsx -expressing neurons, which support the normal execution of copulation in adults by providing 5-HT. Our study highlights the conserved involvement of serotonergic neurons in the control of copulatory mechanisms and the key role of BMP signalling in the formation of a sex-specific circuitry. When successful, male courtship culminates in copulation, yet the neural mechanism underlying copulation has attracted limited attention in biology [1] . Indeed, copulation represents a complex behaviour that consists of coordinated motor acts involving the entire body, and thus requires comprehensive analyses across the molecular, cellular and organismal levels to clarify its neural basis [2] . One of the promising approaches to such investigation would be genetic dissections, which start with isolating mutants with specific defects in copulation. Indeed, mutants with defects of copulation have been identified. coitus interruptus ( coi ) mutant males have shorter copulation durations than wild-type males do [3] . Males of stuck ( sk ) [3] and lingerer ( lig ) [4] mutants often fail in withdrawing their genitalia to terminate copulation. lig mutant males also less frequently attempt copulation despite their normal levels of overall courtship activities [4] . Although these mutations unravelled some of mechanistic elements composing the copulation motor program, they provided fewer insights into the neural basis for copulation. Recent technical advances have allowed the artificial activation and/or inactivation of selected neurons in vivo , opening a route to determination of the circuitries underlying copulation behaviour. This approach led to the identification of pC2l, a dsx -expressing ( dsx [+]) neural cluster in the brain, which plays a role in triggering attempted copulation [5] , as well as eight GABAergic dsx [+] neurons in the abdominal ganglion with roles in regulating the copulation duration [6] . The GABAergic regulation of copulation duration is antagonized by the dopaminergic system in the abdominal ganglion [6] . In addition, insulin-producing cells (IPCs) in the pars intercerebralis, a neurosecretory centre of the insect brain, have been shown to regulate the timing and frequency of attempted copulation; serotonin receptor 1A ( 5-HT 1A ) knockdown in IPCs reduces the latency to abdominal curling and increases the incidence of attempted copulation [7] . 5-HT 1A knockdown in IPCs also shortens the latency to courtship initiation [8] , implying its role as a motivational regulator. Thus, copulation is controlled by a multilayered system that contains, at very least, a brain centre (that is, pC2l) for triggering copulation attempts, a motivational modulator in the brain (that is, IPCs), an abdominal centre for tuning copulation persistence, and an as yet unidentified central pattern generator for the execution of copulation, which is presumably located in the ventral nerve cord (the thoracic and abdominal ganglia [9] ). Starting with the isolation of a mutant named platonic ( plt ), whose males fail to copulate despite vigorous courtship towards a female (reviewed in refs 2 , 10 ), here we identify a hitherto uncovered component of the copulation-controlling dsx [+] neural system, which functions to improve motor performance for copulation by secreting serotonin (5-HT) in the abdominal ganglion. The plt mutation impairs the BMP signalling required for the survival of eight serotonergic interneurons in the abdominal ganglion, and thereby induces copulation defects in mutant males via a 5-HT deficiency. Our results highlight the conserved roles of 5-HT in the regulation of copulation and of BMP signalling in the development of cellular substrates for sex-specific behaviours. plt is an allele of sbb plt homozygotes are semilethal, and exhibit a visible phenotype in the wing vein: the posterior-most wing vein fails to reach the wing margin ( Supplementary Fig. 1 ). The plt mutant line carries an insertion of a ry + -marked P -element at the cytological location 53C. Outcrosses over five generations to a ry − control line led to the segregation of neither the copulation defect nor the wing vein defect from the ry + marker, strongly suggesting that the two apparently unrelated phenotypes are both linked to the same P -element insertion at 53C. Subsequent deficiency mapping verified this idea: two deficiencies, Df(2R)BSC334 and Df(2R)ED3683 , when placed in trans to plt , uncovered the no-copulation phenotype as well as the short-wing vein phenotype in these plt hemizogotes, whereas four other deficiencies, ( Df(2R)BSC335 , Df(2R)BSC399 , Df(2R)BSC483 and Df(2R)Exel7153 ), similarly tested failed to uncover either phenotype ( Fig. 1a ; Supplementary Fig. 1 ). The cytological breakpoints of these deficiencies defined a ∼ 70-kb region within which the genetic sequences responsible for the two phenotypes likely exists ( Fig. 1b ). Searches of the Drosophila genome database revealed a candidate gene annotated to this ∼ 70-kb region, scribbler ( sbb ). Indeed, genetic complementation tests where plt was combined with different sbb mutations demonstrated that plt is allelic to sbb : these heteroallelic mutants manifested both the copulation defect and wing vein defect ( Fig. 1a ; Supplementary Fig. 1 ). plt is thus referred to as sbb plt hereafter. Moreover, inverse PCR of the genomic sequence flanking the mutagenic P -element demonstrated that the P -element was inserted 31-bp downstream of the sbb transcription start site ( Fig. 1c ). As expected, sbb plt hemizygous mutants exhibited a reduction in sbb messenger RNA (mRNA) expression as detected by PCR with reverse transcription ( Supplementary Fig. 2a ). We conclude that the impairment in copulation and wing vein formation in sbb plt resulted from the reduction in sbb expression. 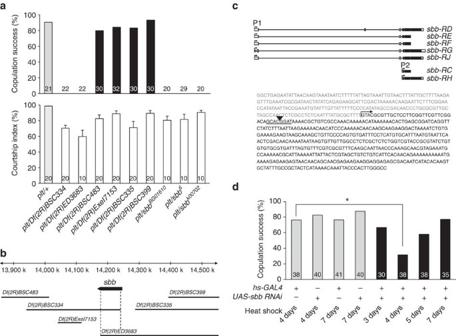Figure 1: Mapping thepltmutation. (a) Courtship activities (lower panel) and copulation success (upper panel) for the indicated mutant and control flies. In the lower panel ofa, the mean±s.e.m. values are shown. (b) Deficiency mapping of thepltmutation onto the genome. The top horizontal bar indicates the physical distance (in kb) relative to thesbbtranscription start site. Thesbb-transcribed region is indicated with an arrow, the direction of which indicates the direction of transcription. The deleted region for each deficiency chromosome is shown below the arrow (horizontal bars). (c) The genomic organization of thesbbgene (upper panel) and the sequence determined by inverse PCR (lower panel). In the upper panel, exons (black boxes: coding regions; open boxes: non-coding regions) and introns (thin horizontal lines) for several transcripts are shown. In the lower panel, the mutagenicP-element insertion site (an inverted triangle), the target sequence of theP-element (underlined) and the transcription start site are indicated. (d) Effect on the copulation rate of developmental timing ofsbbknockdown. The transgenes carried by tested flies are indicated below each bar (+, with the transgene; −, without the transgene). In all graphs, the number of flies examined is indicated below each bar. Ind, statistical differences are evaluated by theχ2-test (*P<0.05). Figure 1: Mapping the plt mutation. ( a ) Courtship activities (lower panel) and copulation success (upper panel) for the indicated mutant and control flies. In the lower panel of a , the mean±s.e.m. values are shown. ( b ) Deficiency mapping of the plt mutation onto the genome. The top horizontal bar indicates the physical distance (in kb) relative to the sbb transcription start site. The sbb -transcribed region is indicated with an arrow, the direction of which indicates the direction of transcription. The deleted region for each deficiency chromosome is shown below the arrow (horizontal bars). ( c ) The genomic organization of the sbb gene (upper panel) and the sequence determined by inverse PCR (lower panel). In the upper panel, exons (black boxes: coding regions; open boxes: non-coding regions) and introns (thin horizontal lines) for several transcripts are shown. In the lower panel, the mutagenic P -element insertion site (an inverted triangle), the target sequence of the P -element (underlined) and the transcription start site are indicated. ( d ) Effect on the copulation rate of developmental timing of sbb knockdown. The transgenes carried by tested flies are indicated below each bar (+, with the transgene; −, without the transgene). In all graphs, the number of flies examined is indicated below each bar. In d , statistical differences are evaluated by the χ 2 -test (* P <0.05). Full size image sbb knockdown in the entire body by the combination of hs-GAL4 and UAS-sbbRNAi induced both the copulation defect and wing vein defect characteristic of sbb plt hemizygous mutants, provided that heat shock was applied at an appropriate time point ( Fig. 1d ; Supplementary Fig. 3 ). PCR with reverse transcription also confirmed that UAS-sbbRNAi can effectively reduce sbb mRNA levels ( Supplementary Fig. 2b ). Interestingly, the most effective time point for heat shock was 4 days after egg laying for both of the phenotypes ( Fig. 1c ; Supplementary Fig. 3 ), indicating that sbb + is required in the larval stage to achieve acquisition of a normal wing vein and normal copulation in the adult fly. This result is compatible with the known developmental roles of Sbb, which functions as a transcription factor in signal transduction downstream of Dpp, a conserved BMP family morphogen [11] , [12] . Neural origin of copulation defects in plt mutants Because our anatomical analysis revealed no obvious structural anomalies in the external genitalia and associated muscles in sbb plt hemizygous mutants ( Supplementary Fig. 4 ), the unsuccessful copulation in these males likely originated from neural malfunction. sbb plt hemizygous mutants gave high courtship indices ( Fig. 1a ; Supplementary Fig. 5a ) displaying wing extension/vibration at high rates ( Supplementary Fig. 5b ), yet having a markedly reduced incidence of licking and attempted copulation ( Supplementary Fig. 5c,d ). These observations support the notion that the copulation defect has a neural origin. Because the major part of the male courtship circuitry has been shown to be composed of neurons that express either or both of the two sex determination genes fruitless ( fru ) and doublesex ( dsx ) [13] , [14] , [15] , we examined the effects of sbb knockdown with UAS-sbbRNAi as driven by fru-GAL4 ( fru GAL4 or fru NP21 ) or dsx-GAL4 ( dsx GAL4 ). In contrast to the partial suppression of copulation success with fru-GAL4 ( Fig. 2a ; Supplementary Fig. 6 ), dsx-GAL4 completely blocked copulation when used to express UAS-sbbRNAi ( Fig. 2b ), with only moderate effects on courtship activities ( Supplementary Fig. 7a,b ). The male flies of all test genotypes actively courted females ( Supplementary Fig. 7a ). Because dsx —unlike neuron-specific fru —is expressed in a wide variety of non-neural as well as neural tissues, we evaluated the relative contribution of non-neural and neural tissues to the sbbRNAi -induced copulation block. When the dsx-GAL4 activity was antagonized by GAL80 expressed selectively in neurons with neuron-specific elav-GAL80 , the copulation block by sbbRNAi was perfectly abrogated ( Fig. 2c ; Supplementary Fig. 8a ), indicating that the no-copulation phenotype is ascribable to the sbb knockdown in dsx -expressing neurons but not non-neural dsx -positive tissues. To further ascertain whether neuronal sbb + is a requirement for normal copulation, dsx -positive glia were excluded from sbbRNAi expression with the aid of repo-GAL80 (the repo promoter is specifically active in glia). This result indicated that sbbRNAi expression via dsx-GAL4 completely blocked copulation irrespective of whether repo-GAL80 was present or not ( Fig. 2d ; Supplementary Fig. 8e ), indicating that glial cells are not involved in this phenotype. 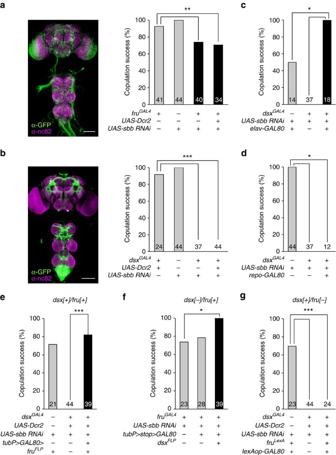Figure 2: Contribution of neurons positive forfruand/ordsxand of glia to the copulation defect in flies withsbbknockdown. Images (left-side panels) of the CNS withfru-positive (a) ordsx-positive (b) neurons and the effect ofsbbknockdown in the respective neurons (right-side panels) on the copulation rate. The genotypes of flies for the histological analysis arew; UAS-mCD8::GFP/+; fruGAL4/+ (a) andw; UAS-mCD8::GFP/+; dsxGAL4/+ (b), respectively. Scale bar, 100 μm. (c,d) Effect of neuron-excluded (c) or glia-excluded (d)sbbknockdown on copulation. (e–g) Effect ofsbbknockdown indsx[+]/fru[+] (e),dsx[−]/fru[+] (f) ordsx[+]/fru[−] (g) on copulation. *P<0.05; **P<0.01; ***P<0.001 by theχ2-test. Data are presented as described in the legend ofFig. 1. Figure 2: Contribution of neurons positive for fru and/or dsx and of glia to the copulation defect in flies with sbb knockdown. Images (left-side panels) of the CNS with fru -positive ( a ) or dsx -positive ( b ) neurons and the effect of sbb knockdown in the respective neurons (right-side panels) on the copulation rate. The genotypes of flies for the histological analysis are w; UAS-mCD8::GFP/+; fru GAL4 /+ ( a ) and w; UAS-mCD8::GFP/+; dsx GAL4 /+ ( b ), respectively. Scale bar, 100 μm. ( c , d ) Effect of neuron-excluded ( c ) or glia-excluded (d) sbb knockdown on copulation. ( e – g ) Effect of sbb knockdown in dsx [+]/ fru [+] ( e ), dsx [−]/ fru [+] ( f ) or dsx [+]/ fru [−] ( g ) on copulation. * P <0.05; ** P <0.01; *** P <0.001 by the χ 2 -test. Data are presented as described in the legend of Fig. 1 . Full size image Some neurons express both dsx and fru ( dsx/fru double-positive cells: dsx [+]/ fru [+]), while others express either dsx or fru ( dsx single-positive cells: dsx [+]/ fru [−]; fru -single-positive cells: dsx [−]/ fru [+]), and the rest express neither of these genes [16] , [17] , [18] . To determine which type of dsx -positive cells requires sbb + for normal copulation, we restricted the action of dsx-GAL4 by expressing GAL80 in a subset of dsx -positive cells using three different intersection strategies. In the first strategy, we used a conditional GAL80 transgene, tubP>GAL80> . Here the two > indicate the FRT sequences, that is, the target of the flippase FLP; the FLP binds to the FRTs flanking GAL80 , thereby excising GAL80 and allowing GAL4 to act. We combined tub>GAL80> with fru FLP , which expresses FLP from the endogenous fru gene promoter, and in this way activated GAL4 only within dsx [+]/ fru [+] cells ( Fig. 2e ). In the second strategy, we used the other conditional GAL80 transgene, tubP>stop>GAL80 , in conjunction with dsx FLP , which expresses FLP via the endogenous dsx gene promoter. Because GAL80 is expressed only when FLP has excised the stop sequence between the tub promoter and the GAL80 -coding region, this transgene allowed us to restrict the activation of GAL4 to only dsx [−]/ fru [+] cells when combined with dsx FLP ( Fig. 2f ). In the third strategy, lexAop-GAL80 was used in the presence of fru LexA . In this case, the LexA transcription factor is produced only in cells where an endogenous fru gene promoter is active, and the resulting LexA binds to lexAop , leading to the generation of GAL80 in these cells, and thus to GAL4 activation only in dsx [+]/ fru [−] cells ( Fig. 2g ). In these three types of experiment, the GAL4 activity was restricted to the cell group as planned, judging from the reporter expression ( Supplementary Fig. 8b–d ). We found that the no-copulation phenotype was attained only when sbbRNAi was expressed in dsx [+]/ fru [−] cells ( Fig. 2e–g ), indicating that dsx single-positive neurons are critically involved in this phenotype. sbb is required in abdominal dsx neurons for normal copulation To further narrow down the neuron groups in which sbb + is required for normal copulation, we restricted GAL4 activity to different fractions of dsx -positive cells using Otd-FLP , which expresses FLP only in the head, using tsh-GAL80 , which prohibits GAL4 activity in the thorax, or selecting GAL4 s that preferentially drive expression in particular groups of neurons that are identified by neurotransmitters. We also tested GAL4 drivers for chemosensory cells ( poxn-GAL4 ) or mechanosensory cells ( ppk-GAL4 ), as these peripheral neurons may guide a male fly (or the male genitalia) to potential copulation targets [19] . When sbb knockdown was targeted to all the central nervous system (CNS) dsx cells except those in the head, the copulation defect was still produced ( Fig. 3a ; Supplementary Fig. 8f ), whereas head-specific sbb knockdown did not impair copulation ( Fig. 3b ; Supplementary Fig. 8g ); these results indicate that the dsx- expressing cells in the brain are not one of the sites at which sbb + may be required for normal copulation. sbb knockdown in dsx -expressing cells in the CNS excluding those in the thorax still induced the copulation defect ( Fig. 3c ; Supplementary Fig. 8h ); this result indicates that the thoracic dsx -expressing cells are not a candidate site for inducing this phenotype. Note, however, that the thoracic dsx neuron cluster called TN2 escaped the action of tsh-GAL80 for an unknown reason, and thus this group of dsx -expressing neurons is not excluded from the candidate sites at which sbb + may function for copulation. In addition, a pair of large dsx neurons in the suboesophageal ganglion (SN) was not amenable to testing due to the lack of tools for its specific manipulation. These results collectively indicate that the dsx -expressing neurons in the non-thoracic ventral nerve cord (VNC), dsx -positive TN2 and dsx -positive SN remain as candidate cells. Peripheral mechano- and chemo-sensory neurons were judged not to make a large contribution to the no-copulation phenotype induced by sbb knockdown ( Supplementary Fig. 9 ). Eight neurotransmitter-defined GAL4 s representing six neurotransmitter species were tested in conjunction with dsx FLP and tubP>GAL80> : acetylcholine ( Cha-GAL4 ), octopamine ( Tdc2-GAL4 ), dopamine ( TH-GAL4 ), 5-HT ( Trh-GAL4 ), L -glutamate ( Vglut 0k371 -GAL4 and Vglut-GAL4 on X) and GABA (γ-aminobutyric acid; GAD-GAL4 on 2nd and GAD-GAL4 on 3rd). The most striking inhibition of copulation was observed when sbbRNAi was expressed under the control of Trh-GAL4 or GAD-GAL4 , although Cha-GAL4 , TH-GAL4 and Vglut-GAL4 also yielded significant reductions in copulation success when used as drivers for sbbRNAi expression ( Fig. 3d ; Supplementary Figs 7c, 10 and 11 ). For further functional analysis, we used Trh-GAL4 , which drove expression in a relatively small number of VNC cells compared with the other seven GAL4 s, each of which yielded expression in hundreds of VNC cells, yet Trh-GAL4 was the most effective of the GAL4 drivers of sbbRNAi expression tested in terms of inhibiting copulation. We assumed that a small number of Trh-GAL4 -positive neurons may have a decisive effect on copulation success. Although Trh-GAL4 was used with the intention of labelling and manipulating serotonergic cells, the putative cis -region of a gene fused with GAL4 does not necessarily recapitulate the endogenous expression of the gene in transformant flies. In fact, two GAD-GAL4 lines used in this study revealed noticeably different expression patterns of a reporter in the CNS ( Fig. 3e,f ). We therefore performed double staining of the CNS for the expression of the Trh - GAL4 -driven reporter and the immunoreactivity to an anti-5-HT antibody, and found that the Trh-GAL4 expression coincides, in principle, with the anti-5-HT immunoreactivity ( Supplementary Fig. 10c ). However, there were also discrepancies between the Trh-GAL4 expression and localization of anti-5-HT immunoreactivity. For example, ‘ tsh-GAL80 -resistant’ TN2 were positive for Trh-GAL4 but negative for 5-HT ( Supplementary Fig. 10c ). In addition, TN2 and ‘ Otd-FLP -insensitive’ SN were labelled by two other GAL4 s, GAD-GAL4 and Vglut-GAL4 ( Fig. 3e,h ; Supplementary Fig. 10a,b ), although both TN2 and SN were negative for anti-GABA immunoreactivity ( Supplementary Fig. 11a,b ). We were unsuccessful in staining the VNC with antibodies against L -glutamate or Vglut. Next, therefore, we attempted to elucidate a key role of the serotonergic neurons in successful copulation using an experiment to examine the effect of deprivation and supplementation of 5-HT on copulation (see below). It is noteworthy that only a total of eight dsx -expressing cells were labelled by the intersection of Trh-GAL4 and dsx FLP ( Fig. 3g ), even though sbbRNAi expression in these eight cells resulted in a marked reduction in copulation success ( Fig. 3d ). We therefore considered that the Trh-GAL4 -positive dsx neurons may be promising candidates for the site of sbb + action in the control of copulation, although we cannot completely exclude the possibility that sbb + activity is also required in other cells, including SN and TN2, for normal copulation. 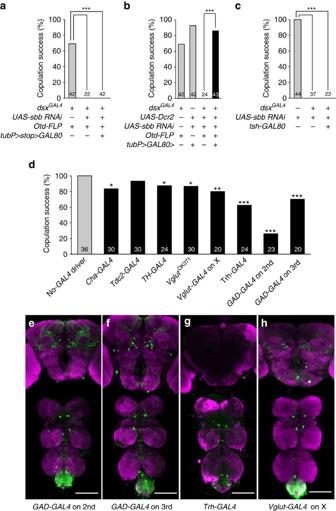Figure 3: Effect ofsbbknockdown in subsets ofdsxneurons as defined by their body region or by the transmitters they synthesize. Effect of head-excluded (a), head-specific (b) and thorax-excludedsbbknockdown indsx-expressing neurons (c) on copulation. (d) Comparisons ofGAL4s defined by transmitters in terms of their effect on copulation when used to driveUAS-sbbRNAionly indsx-expressing cells by means oftubP>GAL80>anddsxFLP. (e–h) Images ofdsxneurons that expressGAD-GAL4on 2nd (e),GAD-GAL4on 3rd (f), orTrh-GAL4(g) orVglut-GAL4on X (h). The genotypes of flies werew; GAD-GAL4 on 2nd/UAS>stop>mCD8::GFP; dsxFLP/+ (e),w; UAS>stop>mCD8::GFP/+; dsxFLP/GAD-GAL4on 3rd (f),w; Trh-GAL4/UAS>stop>mCD8::GFP; dsxFLP/+ (g) andVglut-GAL4on X; UAS>stop>mCD8::GFP/+; dsxFLP/+ (h), respectively. *P=0.05; **P=0.01; ***P=0.001 Scale bar, 100 μm. Figure 3: Effect of sbb knockdown in subsets of dsx neurons as defined by their body region or by the transmitters they synthesize. Effect of head-excluded ( a ), head-specific ( b ) and thorax-excluded sbb knockdown in dsx -expressing neurons ( c ) on copulation. ( d ) Comparisons of GAL4 s defined by transmitters in terms of their effect on copulation when used to drive UAS-sbbRNAi only in dsx -expressing cells by means of tubP>GAL80> and dsx FLP . ( e – h ) Images of dsx neurons that express GAD-GAL4 on 2nd ( e ), GAD-GAL4 on 3rd ( f ), or Trh-GAL4 ( g ) or Vglut-GAL4 on X ( h ). The genotypes of flies were w; GAD-GAL4 on 2nd/UAS>stop>mCD8::GFP; dsx FLP /+ ( e ), w; UAS>stop>mCD8::GFP/+; dsx FLP /GAD-GAL4 on 3rd ( f ), w; Trh-GAL4/UAS>stop>mCD8::GFP; dsx FLP /+ ( g ) and Vglut-GAL4 on X ; UAS>stop>mCD8::GFP/+; dsx FLP /+ ( h ), respectively. * P =0.05; ** P =0.01; *** P =0.001 Scale bar, 100 μm. Full size image Serotonergic neuronal death results in plt copulation defects An obvious question here is why the partial loss of function in sbb at the larval stage impairs copulation performance in the adult stage. Immunostaining of Trh-GAL4 -positive dsx -expressing neurons in flies that also carried UAS-sbbRNAi revealed that nearly half of these cells were lost by sbb knockdown (3.6±1.2, n =5 in sbb knockdown versus 7.7±0.7, n =9 in the control; Fig. 4a,b ). Different sets of cells seemed to be lost in different flies with sbb knockdown. Thus, it is plausible that the presence of eight serotonergic dsx -positive neurons in the abdominal ganglion is essential for normal copulation to occur. Indeed, double staining for Trh-GAL4 -driven mCD8::GFP and 5-HT immunoreactivity in the presence of dsx FLP highlighted these eight Trh -positive dsx neurons ( Fig. 4c ; Supplementary Fig. 10c ), indicating that these cells express 5-HT. We consider that sbb + is required in the serotonergic dsx -positive cells for their normal development. Failures in this process likely trigger degeneration of some of these cells with a consequence of 5-HT deficiency. Careful fluorescent microscopic examinations of these eight neurons as labelled by mCD8::GFP did not reveal peripheral axons, indicating that they are all interneurons. 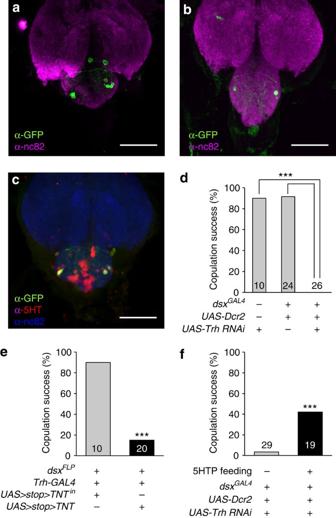Figure 4: Roles of serotonergicdsxneurons and 5-HT in copulation. Images ofTrh-GAL4-positivedsxneurons in the abdominal ganglion in male flies without (a) and with (b)sbbknockdown. The genotypes of flies werew; Trh-GAL4/UAS>stop>mCD8::GFP; dsxFLP/+ (a) andw; Trh-GAL4/UAS-sbbRNAi tubP>GAL80>; dsxFLP/UAS>stop>mCD8::GFP(b), respectively. Scale bar, 50 μm. (c)Trh-GAL4-positivedsxneurons are immunopositive for an anti-5-HT antibody. Scale bar, 50 μm. (d)Trhknockdown indsx-positive neurons completely blocks copulation. (e) Block of synaptic outputs from serotonergicdsxneurons byTNTinhibits copulation. InactiveTNT(TNTin) has no effect. (f) Copulation defects are rescued by feeding adults on 5-HTP-supplemented foods. 5-HTP was administered at 100 mM according to ref.20. The mean±s.e.m. and the number of flies examined are shown. ***P<0.001 by theχ2-test. Figure 4: Roles of serotonergic dsx neurons and 5-HT in copulation. Images of Trh-GAL4 -positive dsx neurons in the abdominal ganglion in male flies without ( a ) and with ( b ) sbb knockdown. The genotypes of flies were w; Trh-GAL4/UAS>stop>mCD8::GFP; dsx FLP /+ ( a ) and w; Trh-GAL4/UAS-sbbRNAi tubP>GAL80>; dsx FLP /UAS>stop>mCD8::GFP ( b ), respectively. Scale bar, 50 μm. ( c ) Trh-GAL4 -positive dsx neurons are immunopositive for an anti-5-HT antibody. Scale bar, 50 μm. ( d ) Trh knockdown in dsx -positive neurons completely blocks copulation. ( e ) Block of synaptic outputs from serotonergic dsx neurons by TNT inhibits copulation. Inactive TNT ( TNT in ) has no effect. ( f ) Copulation defects are rescued by feeding adults on 5-HTP-supplemented foods. 5-HTP was administered at 100 mM according to ref. 20 . The mean±s.e.m. and the number of flies examined are shown. *** P <0.001 by the χ 2 -test. Full size image To evaluate the importance of 5-HT in dsx -expressing cells in male copulation performance, we knocked Trh down in these cells, which exhibited a reduction in trh mRNA expression and a decrease in the number of cells with detectable 5-HT immunoreactivity ( Supplementary Fig. 12 ). Intriguingly, Trh knockdown in all dsx- expressing cells completely blocked copulation ( Fig. 4d ), reminiscent of the sbb plt mutant phenotype. Block of synaptic outputs from these neurons with Tetanus toxin light chain (TNT) also inhibited copulation ( Fig. 4e ; Supplementary Fig. 7e ). In contrast, activation via dTrpA1 of the same set of neurons was without effect: copulation success in the presence of a female was not increased (75% at 19 °C, 71% at 32 °C; n =24) nor did a solitary male display motions associated with copulation. This might mean that 5-HT secreted by these neurons gates execution of copulation when the released dose exceeds a threshold, but elicits no further effect at higher doses beyond the threshold. To determine whether 5-HT is necessary for executing copulation at the adult stage or for normal development of neural components, we examined the effect of supplementing foods with the 5-HT precursor 5-hydroxytriptophan (5-HTP) after adult emergence [20] . When flies with Trh knockdown in dsx -expressing cells were fed with 5-HTP only at the adult stage, the emerged adult males exhibited higher copulation success ( Fig. 4f ; Supplementary Fig. 7d ), accompanied by an increase in the number of cells with detectable 5-HT immunoreactivity in dsx-GAL4 -positive cells ( Supplementary Fig. 12 ). These results demonstrate that 5-HT functions in the control of copulation at the adult stage. Overall, our results indicate that sbb + at the larval stage supports the survival of a subset of dsx -positive VNC neurons that produce 5-HT, which is essential for copulation to occur at the adult stage. The sbb gene encodes C2H2-type zinc-finger proteins that function downstream of the major morphogen Dpp [11] , [12] , and thus plays roles in a variety of cellular events, including those pivotal for neural developments such as axon guidance [21] . In this paper, we presented evidence that sbb expression is essential for the survival of a subset of serotonergic neurons, which are lost if sbb is lost at the critical period before imaginal metamorphosis. A notable analogy to the neuronal loss due to sbb loss observed in this study is the massive cell death reported in the developing wing disc induced by mutations in optomoter-blind ( omb ), a gene encoding a transcription factor also acting downstream of Dpp; Omb transcriptionally represses the Dpp receptor gene thickvein ( tkv ), and failure in this repression results in tkv upregulation, which ultimately causes cell death [22] . Importantly, Omb requires Sbb to repress tkv expression in the larval wing disc [22] . We postulate that Sbb similarly functions to shut down Dpp signalling in the serotonergic dsx neurons at a defined time window before the imaginal metamorphosis for proper differentiation of these neurons. The BMP family proteins to which Dpp belongs are conserved across phyla, thereby playing central roles in a variety of morphogenetic events, including sexual character development. For example, the formation of papillary processes in the anal fin, a masculine sexual characteristic in Medaka fish, is induced by androgen via the enhancement of BMP7 expression [23] . Thus, there may exist interesting parallels between vertebrate and invertebrate development in that BMP and the sex-determinant machinery coordinate to specify male-specific characteristics with roles in mating. In contrast to the developmental role of sbb + , 5-HT produced by Trh -positive dsx neurons in the VNC is required for the control of copulation in the adult stage. The exact role of serotonergic dsx neurons in the VNC in the control of copulatory mechanisms remains to be clarified. Higher-resolution motion recordings of a fly attempting copulation might help in detecting subtle yet critical changes in the specific movements of abdominal structures in sbb mutant males. Although in this study we focused on VNC neurons, it has been demonstrated that activities in a specific cluster of dsx single-positive neurons called pC2l (ref. 24 ) in the brain trigger copulation behaviour [5] . Also, there is evidence of the involvement of the brain serotonergic system in regulating motivation to copulate [25] , [26] . These brain neurons appear to turn ON and OFF, via as yet unidentified descending neurons, the VNC motor centre for the control of copulation, whose development and function are likely regulated by the Trh-GAL4 -positive dsx neurons we found in this study. Once initiated, copulation seems to be accomplished by ‘copulation-executor’ VNC neurons, which may also determine the duration of copulation. Some such VNC neuron groups that affect the copulation duration have been identified, that is, fru -positive serotonergic motoneurons innervating internal reproductive organs [27] , corazonin-expressing interneurons and their associated downstream serotonergic motoneurons [28] , and dsx -expressing GABAergic interneurons [6] . A factor affecting the copulation duration is the level of ‘persistence’, which can be assessed by the effectiveness of a disturbance stimulus to curtail ongoing copulation. An interrupting mating test, performed to measure the ease with which males could be separated from females upon 60-s vortexing, previously revealed that a disturbance stimulus applied during the first 5-min period after the copulation initiation is least effective in forcing a pair to dissociate, and thus that the level of persistence is highest over that time period [3] . The persistence level then gradually decreases over the subsequent 10–15 min, and the copulation ultimately terminates without any disturbance [3] . A later work suggested that the copulation persistence is negatively regulated by the eight dsx -positive GABAergic interneurons in the VNC and positively regulated by a dopaminergic system [6] . Our manipulation of serotonergic neurons in the VNC, in contrast, had no discernible impact on persistence of copulation, once the flies started copulation. These considerations give rise to the supposition that copulation is controlled by a multilayered circuitry in which dsx -expressing and/or aminergic neurons predominate. 5-HT also plays key roles in the central and peripheral systems for control of copulation in humans and other vertebrates [29] , and thus highlights interesting evolutionary parallels across the animal kingdom. Drosophila stocks Flies were reared on cornmeal-yeast medium under a 12:12 light:dark cycle at 25 °C, except for those carrying a transgene for RNA interference (RNAi), which were raised at 29 °C. For the heat-shock induction of sbb double-stranded RNA ( Fig. 1d ), larvae or pupae in food vials were exposed to heat shock of 37 °C for 45 min or 1 h at the indicated developmental timing. The following strains were established, or kept as lab stocks in our laboratory: the wild-type Canton-S , +; plt/SM1; ry 506 , elav C155 -GAL4 , N630 hs-GAL4 , w; UAS-mCD8::GFP , w; UAS-GFPNZ and w;; fru NP21 /TM3 Ser . yw; FRT42 sbb 6 /CyO Act-GFP , yw; sbb k00702 /CyO and P{GT1}sbb BG01610 /CyO were the kind gifts from Tetsuya Tabata (University of Tokyo) [12] . fru GAL4 , fru FLP , UAS>stop>mCD8::GFP, UAS>stop>TNT, UAS>stop>TNT in and UAS>stop>dTrpA1 were the kind gift from Barry J. Dickson (HHMI-Janelia Farm Research Campus) [30] , [31] . dsx GAL4 , dsx FLP and elav-GAL80 were the kind gifts from Stephen F. Goodwin (University of Oxford) [17] , [32] . repo-GAL80 was the kind gift from Leslie B. Vosshall (Rockefeller University) [6] . fru LexA was the kind gift from Bruce S. Baker (HHMI-Janelia Farm Research Campus) [33] . Otd-FLP was the kind gift from David J. Anderson (California Institute of Technology) [34] . tsh-GAL80 was the kind gift from Julie Simpson (HHMI-Janelia Farm Research Campus). w;; poxn-GAL4-14-1-7 , UAS-mCD8::GFP was a gift from Ken-ichi Kimura (Hokkaido University of Education). w, ppk-GAL4 was the kind gift from Kazuo Emoto (University of Tokyo). w;; GAD-GAL4 on 3rd was the kind gift from Yuh Nung Jan (University of California at San Francisco) [35] . The following strains were obtained from the Bloomington Stock Center: w 1118 ; Df(2R)ED3610/CyO (#9066) , w 1118 ; Df(2R)BSC334/CyO (#24358) , w 1118 ; Df(2R)ED3683/SM6a (#8918) , w 1118 ; Df(2R)BSC335/CyO (#24359) , w 1118 ; Df(2R)Exel7153/CyO (#7893) , w 1118 ; Df(2R)BSC399/CyO (#24423) , w 1118 ; Df(2R)BSC483/CyO (#24987) , w; Tdc2-GAL4 (#9313), w;; TH-GAL4 (#8848), Vglut-GAL4 on X (#24635), w 1118 ; Vglut OK371 -GAL4 (II) (#26160) , w; Cha-GAL4, UAS-GFP (#6793) , w; Trh-GAL4 (#38388) , w; GAD-GAL4 on 2nd (#51630) , w; UAS-Dcr2 (#24650) , w;;UAS-Dcr2 (#24651) , tubP>GAL80>; Bl/CyO; TM2/TM6 (#38879) , w; tubP>GAL80>/CyO; TM2/TM6 (#38880) , w; Sp/CyO; tubP>GAL80>/TM6B (#38881) , w; tubP>stop>GAL80>; MKRS/TM6 (#38878) , w; wg Sp-1 /CyO; tubP>stop>GAL80 (#39213), w; UAS>stop>mCD8::GFP; UAS>stop>mCD8::GFP (#30032) , w;; LexAop-GAL80 (#32213) and UAS-Trh-RNAi (#25842). The w 1118 ;UAS-sbbRNAi (#41845) strain was obtained from the Vienna Drosophila Resource Center. Behavioural assays The virgin males and females were collected at eclosion. Males were placed singly in food vials, while 10 females were placed together in single food vials. They were kept at 25 °C until being subjected to behavioural assays. For the 5-HTP treatment ( Fig. 4f ), virgin males carrying both Trh-RNAi and dsx-GAL4 were collected upon emergence, and kept singly with food containing 100 mM 5-HTP [20] . Control flies were fed on normal food without 5-HTP throughout the larval and adult stages. The flies were kept at 25 °C until behavioural assays. Behavioural assays were carried out on males aged 5–7 days after eclosion. The male was placed in a small chamber (0.8 cm in diameter, 0.3 cm in height) with a wild-type virgin female (5–7 days after eclosion). The mating behaviour was recorded for 60 min by a charge-coupled device camera (WAT-221S, Watec, Japan). The courtship activity was quantified by the courtship index, which was defined as the proportion of time a male spent for courtship within an observation period (see below). Actions considered to be elements of courtship included: orientation, following, tapping, wing extension, licking and attempted copulation. The observation period started just after the introduction of the virgin female into the observation chamber. The observation period for the courtship index calculation was 10 min, or until the time when copulation started within the 10 min observation period. The mating success was calculated as the number of pairs that copulated during the observation period (60 min) divided by the number of total pairs observed. In every experiment, we chose a sample size similar to that adopted in preceding works so as to ensure adequate power to detect a meaningful difference among the data sets. The experiments were replicated by at least two different researchers. The statistical analyses were carried out by the Kruskal–Wallis test with Steel–Dwass multiple pair-wise post hoc comparisons for the courtship index, or by the χ 2 -test for the mating success. Immunohistochemistry The CNS was dissected from flies in PBS, and fixed in 4% paraformaldehyde in PBS for 60 min. Immunostaining was carried out as described previously [16] , using the following antibodies at the indicated dilutions: rabbit anti-GABA diluted at 1:500 (Sigma), rabbit anti-5-HT at 1:500 (Sigma), chicken anti-GFP at 1:1,000 (Abcam), rabbit polyclonal anti-GFP at 1:1,000 (Molecular Probes) and mouse monoclonal nc82 at 1:20 (DSHB, University of Iowa, IA). The secondary antibodies used were as follows: Alexa647-conjugated goat anti-mouse IgG at 1:200, Alexa546-conjugated goat anti-rabbit IgG at 1:200, Alexa488-conjugated goat anti-chicken IgG at 1:200, Alexa488-conjugated goat anti-rabbit IgG at 1:200 and Alexa546-conjugated goat anti-mouse IgG at 1:200 (all from Invitrogen). Stacks of optical sections were obtained with a Zeiss LSM 510 META confocal microscope and were processed with Image J software. Data availability The authors declare that the data supporting the findings of this study are available within the article (and its Supplementary Information files), or available from the authors on request. How to cite this article: Yilmazer, Y. B. et al . Serotonergic neuronal death and concomitant serotonin deficiency curb copulation ability of Drosophila platonic mutants. Nat. Commun. 7, 13792 doi: 10.1038/ncomms13792 (2016). Publisher's note: Springer Nature remains neutral with regard to jurisdictional claims in published maps and institutional affiliations.